The built-in electric field across FeN/Fe3N interface for efficient electrochemical reduction of CO2to CO Nanostructured metal-nitrides have attracted tremendous interest as a new generation of catalysts for electroreduction of CO 2 , but these structures have limited activity and stability in the reduction condition. Herein, we report a method of fabricating FeN/Fe 3 N nanoparticles with FeN/Fe 3 N interface exposed on the NP surface for efficient electrochemical CO 2 reduction reaction (CO 2 RR). The FeN/Fe 3 N interface is populated with Fe−N 4 and Fe−N 2 coordination sites respectively that show the desired catalysis synergy to enhance the reduction of CO 2 to CO. The CO Faraday efficiency reaches 98% at −0.4 V vs. reversible hydrogen electrode, and the FE stays stable from −0.4 to −0.9 V during the 100 h electrolysis time period. This FeN/Fe 3 N synergy arises from electron transfer from Fe 3 N to FeN and the preferred CO 2 adsorption and reduction to *COOH on FeN. Our study demonstrates a reliable interface control strategy to improve catalytic efficiency of the Fe–N structure for CO 2 RR. Converting CO 2 back to carbon (C)-based chemicals/fuels is a critical step en route to realizing green environment and energy sustainability [1] , [2] , [3] , [4] , [5] . CO 2 can in principle be reduced to active forms of C-products, but the activated CO 2 intermediates tend to undergo different reaction pathways, making it difficult to efficiently control the reaction selectivity [6] , [7] , [8] . Recently, the electrochemical CO 2 reduction reaction (CO 2 RR) has been studied extensively due to its appealing potential to reduce CO 2 with renewable electricity [9] , [10] . The center of these studies lies in the development of robust catalysts to lower the reduction overpotentials and to direct reaction pathways towards specific C-products. Among all possible products generated from the CO 2 RR, CO is an important precursor that is widely used for preparing other chemicals and fuels [11] , [12] , [13] . 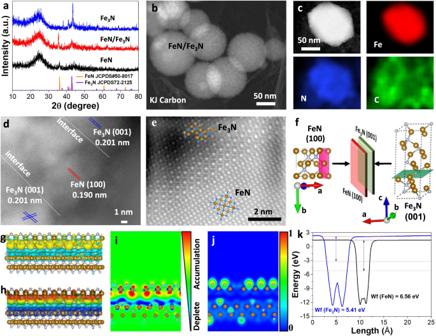Fig. 1: Fe-N NP characterization. aXRD patterns of FeN, FeN/Fe3N, and Fe3N NPs.bSTEM image of FeN/Fe3N NPs.cElemental mapping of Fe, N and C of a single FeN/Fe3N NP.dHRTEM image of FeN/Fe3N NPs showing the interface between FeN and Fe3N domains.eHRHAADF-STEM image of the FeN/Fe3N interface.fSchematic illustration of the FeN/Fe3N interface formed between FeN (100) and Fe3N (001).g3D electron density difference distributions at the FeN/Fe3N interface.hThe electrostatic potential of the FeN/Fe3N interface.iThe electron localization function of the FeN/Fe3N interface.j2D cross-section of electron density difference at the FeN/Fe3N interface.kThe calculated work functions (Wf) of FeN and Fe3N. In the CO 2 RR process, CO is produced via two electron reduction of CO 2 [14] , [15] , and this reaction can be catalyzed by many different catalysts, including not only noble metals (Au, Ag, and Pd) [16] , but also non-noble metals (Cu, CuIn alloys) [17] , [18] , and metal−N 4 (M−N 4 ) complex structures [19] , [20] , [21] , as summarized in Supplementary Table 1 . The M−N 4 structures, especially Ni−N- and Fe−N-based structures, have attracted particular interest as a class of catalysts for CO 2 RR to CO due to increased electron conductivity with decreased band gap of M−N 4 structures and intensive bonding interactions between *COOH intermediates and metal centers, thus lowering the overall reaction barriers and promoting CO generation. However, the Ni−N-complex catalysis is limited by slow kinetics of CO 2 + H + + e − → *COOH and weak *H binding for necessary hydrogenation steps, while the Fe−N-complex catalysis is hindered by the strong *CO and *H binding to the Fe−N sites, which prevent CO from being released as a gas form, or from being further activated for the following hydrogenation steps [20] , [22] , [23] , [24] . Therefore, it is important to stabilize the chemical environment of metal-N-catalysts and to optimize their catalysis towards hydrogenation or desorption of CO at low overpotentials for successful CO 2 RR. Here, we report a strategy to improve Fe−N catalysis efficiency for CO 2 RR. The catalyst is based on FeN/Fe 3 N heterostructure nanoparticles (NPs) in which Fe is coordinated by 4 N’s and 2 N’s respectively, forming a unique Fe−N 4 /Fe−N 2 interface on the NP surface. This interface offers the desired synergetic effect on CO 2 adsorption on FeN, and electron transfer from Fe 3 N to FeN, enhancing the CO 2 reduction to CO. In the CO 2 -saturated 0.5 M KHCO 3 solution, the catalyst shows a high CO Faradaic efficiency (FE) of 98% at −0.4 V (vs. RHE) without noticeable efficiency change in the 100 h electrolysis test between −0.4 V and −0.9 V. The catalysis produces CO with a high single-pass conversion rate up to 56%, which is unprecedented. Our study presents an interface design strategy for improving CO 2 RR catalysis efficiency. The FeN/Fe 3 N NPs were prepared via nitridation of an Fe salt that was pre-deposited on the commercial Ketjen (KJ) carbon support. In the process, Fe(NO 3 ) 3 ·9H 2 O urea and carbon support were mixed in water under ultrasonication, separated from the solution, washed with ethanol and deionized (DI) water, and dried under vacuum at 60 °C. The dried sample was then annealed under a flow of ammonia gas at different temperatures (300, 500, and 700 °C) to initiate iron nitride NP formation (see details in methods, and Supplementary Fig. 1 ). The NP crystal structure was analyzed by powder X-ray diffraction (XRD). Annealing at 300 °C led to the formation of FeN NPs with a cubic structure (space group F-43m, JCPDS No. 50 − 8017, a = b = c = 4.307 Å), annealing at 700 °C gave Fe 3 N NPs with a hexagonal structure (space group of P312, JCPDS No. 72 − 2125, a = b = 4.789 Å, c = 4.710 Å), while annealing at 500 °C yielded FeN/Fe 3 N NPs (Fig. 1a ). The FeN/Fe 3 N, FeN, and Fe 3 N NPs are spherical and uniform, as shown in the scanning transmission electron microscopy (STEM) image (Fig. 1b and Supplementary Fig. 2 ). STEM mapping images display the similar Fe and N elements distribution across each FeN/Fe 3 N (Fig. 1c ), FeN and Fe 3 N NP (Supplementary Fig. 2 ). The high-resolution TEM (HRTEM) image of the FeN/Fe 3 N NPs (Fig. 1d ) shows clear FeN/Fe 3 N domains and interfaces with the lattice mismatch at 5.12% (detail in Methods). The detailed analysis of the FeN/Fe 3 N area by high resolution high-angle annular dark field aberration-corrected STEM (HAADF-STEM) reveals that the interface is created by the junction between cubic FeN and hexagonal Fe 3 N (Fig. 1e ) with obvious atomic dislocation and two distinct diffraction spots at the junction (Supplementary Fig. 3 ). Away from the junction, the FeN (Supplementary Fig. 4 ) and Fe 3 N (Supplementary Fig. 5 ) regions are in single crystalline, showing no atomic dislocation. Additionally, the fast Fourier transform (FFT) images (Supplementary Fig. 6 ) of different regions in Fig. 1e further confirm the FeN/Fe 3 N interface is formed with slightly distorted cubic and hexagonal structure. The N 2 and CO 2 adsorption ability of the Fe–N structures were measured by the Brunner–Emmet–Teller (BET) method under N 2 and CO 2 atmosphere (Supplementary Fig. 7 ). The FeN/Fe 3 N structure adsorbs more N 2 (736.1 m 2 g −1 ) than the FeN (314.5 m 2 g −1 ) and Fe 3 N (586.0 m 2 g −1 ) ones, while the FeN structure adsorbs more CO 2 (25.8 cm 2 g −1 ) than the FeN/Fe 3 N (24.7 cm 2 g −1 ) and Fe 3 N (11.2 cm 2 g −1 ) ones, suggesting that the FeN/Fe 3 N structure may be more porous, but it is the presence of the Fe–N 4 coordination sites in the FeN structure that shows higher CO 2 adsorption power. Fig. 1: Fe-N NP characterization. a XRD patterns of FeN, FeN/Fe 3 N, and Fe 3 N NPs. b STEM image of FeN/Fe 3 N NPs. c Elemental mapping of Fe, N and C of a single FeN/Fe 3 N NP. d HRTEM image of FeN/Fe 3 N NPs showing the interface between FeN and Fe 3 N domains. e HRHAADF-STEM image of the FeN/Fe 3 N interface. f Schematic illustration of the FeN/Fe 3 N interface formed between FeN (100) and Fe 3 N (001). g 3D electron density difference distributions at the FeN/Fe 3 N interface. h The electrostatic potential of the FeN/Fe 3 N interface. i The electron localization function of the FeN/Fe 3 N interface. j 2D cross-section of electron density difference at the FeN/Fe 3 N interface. k The calculated work functions (W f ) of FeN and Fe 3 N. Full size image We used the density functional theory (DFT) to further investigate the FeN/Fe 3 N structure (Fig. 1f–k ). The (100) planes of FeN (pink) (interplanar distance 4.230 Å) and (001) planes of Fe 3 N (green) (interplanar distance 4.656 Å) match well to form the junction (Fig. 1f ). We calculated electron density difference distributions [25] between the FeN/Fe 3 N interface. As shown in Fig. 1g , the electron clouds around N and Fe in the FeN region (yellow) are much more enriched than that in the Fe 3 N region (blue), indicating the electron transfer from Fe 3 N to FeN. Due to this electron transfer, the FeN region becomes nucleophilic (Fig. 1h red and yellow region), while the Fe 3 N region is electrophilic (Fig. 1h blue region). The distribution of electrons across the interface structure was studied by 2D electron density distribution and electron location function, as shown in Fig. 1i, j . More electrons are localized over the FeN domain than over the Fe 3 N one. This is further supported by the calculated electrostatic potential [26] (Fig. 1k ) with the work function of FeN at 6.56 eV and Fe 3 N at 5.41 eV. Therefore, in the FeN/Fe 3 N interface structure, there exists a built-in electric field from Fe 3 N to FeN. The Fe K-edge of the extended X-ray absorption fine structure spectroscopy (EXAFS) of the Fe 3 N/FeN NPs show the increased energy of the fingerprint peak from Fe 3 N (7096.8 eV) to FeN (7108.5 eV) (Fig. 2a ), indicating the Fe valence state change from +1 in Fe 3 N to +3 in FeN [27] , [28] . There is also a fingerprint peak (7106.4 eV) that is located in the middle of the Fe 3 N and FeN, implying that the Fe valence in the FeN/Fe 3 N interface region is between +1 and +3. The pre-edge peaks at 7089.7 and 7088.2 eV are from Fe−N 4 with tetrahedral coordination (Fe Td , Insert in Fig. 2a right) [29] , [30] , not the octahedral coordination (Fe Oct , Insert in Fig. 2a left) in the Fe 3 N structure [31] . The Fourier transform k 3 -weighted EXAFS (FT-EXAFS) spectra in Fig. 2b (R space) show main peaks in the range from 1 to 3 Å. With more N binding to Fe, the Fe–Fe distance gets longer and longer (in the 2 − 3 Å range), but the Fe–N distance is shorter (in the 1–2 Å range), showing a double peak for the Fe Oct − N (in the Fe 3 N structure) and a broad peak for the Fe Td − N (in the FeN structure). The main peak at 2.33 Å in the Fe 3 N spectrum is close to the Fe−Fe bond (2.23 Å) measured from the Fe foil. Fittings of the FeN (Supplementary Fig. 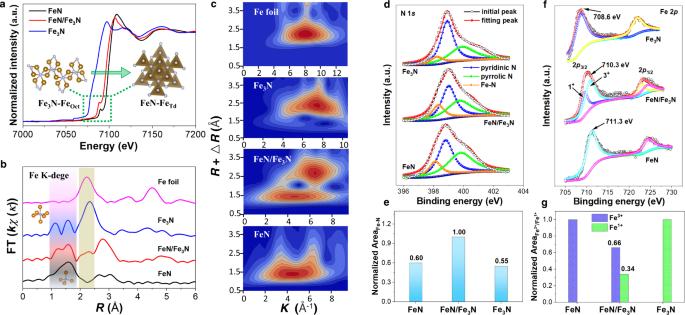Fig. 2: Fe-N NP coordination and electron structure characterization. aThe normalized Fe K-edge EXAFS spectra. Inset: the local FeN structure showing tetrahedral coordination (right) and Fe3N structure showing octahedral coordination (left).bFe K-edge FT-EXAFS in R space andcwavelet transforms for the k3-weighted EXAFS signals for FeN, FeN/Fe3N, Fe3N, and Fe foil.dThe N 1sXPS spectra,ethe normalized area of Fe–N bond,fthe Fe 2pXPS spectra, andgthe normalized area of Fe3+/Fe1+for FeN, FeN/Fe3N, and Fe3N, respectively. 8 and Supplementary Table 2 ) and Fe 3 N (Supplementary Fig. 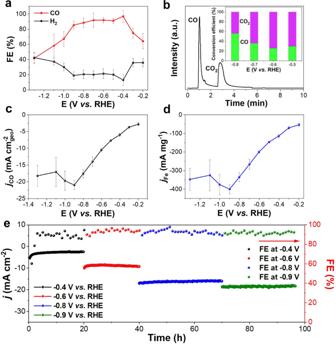Fig. 3: CO2RR performance of the FeN/Fe3N catalyst. aReduction potential dependent FEs of CO and H2.bGC spectrum of the gas products upon a single pass CO2conversion (Inset: reduction potential dependent CO2conversion to CO).cCO partial current density anddcorresponding mass activity.eCO2RR current density and CO FE changes at different reduction potentials over different electrolysis times. Error bars ina–drepresent the standard deviation of three independent measurements. 9 and Supplementary Table 3 ) spectra suggest that Fe has a coordination number (CN) of 3.92 and 1.40 respectively. The FeN/Fe 3 N structure shows more complex peaks in the R-space with Fe−N 4 peak at 1.60 Å and Fe–N 2 peak at 2.33 Å. The corresponding fitting gives the CN of 3.60 for the Fe–N 4 and 1.80 for the Fe–N 2 structure (Supplementary Fig. 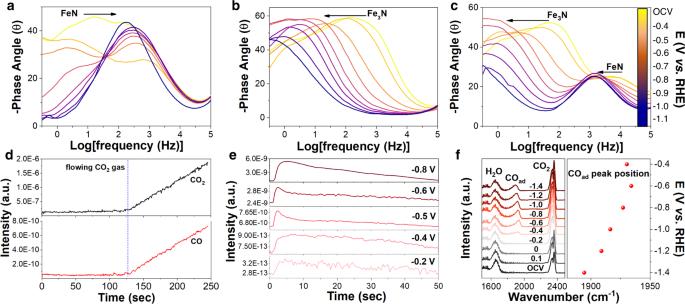Fig. 4: In situ spectroscopic studies of Fe-N catalysts and CO2RR. a–cBode phase plots of FeNa, Fe3Nb, and FeN/Fe3Ncat different reduction potentials. In situ DEMS plots showing the increased presence of CO with increased flowing CO2gasdand CO signal under different potentialseof the FeN/Fe3N-catalyzed CO2RR.fThe in situ SEIR spectra of the FeN/Fe3N for CO2RR. 10 and Supplementary Table 4 ). The Fe–N structures were further analyzed by wavelet transform of the EXAFS [26] . As shown in Fig. 2c , both FeN and FeN/Fe 3 N have the K values centered around 4.8 Å −1 , while those values from Fe 3 N and FeN/Fe 3 N locate at 6.5 (FeN/Fe 3 N) and 7.5 Å −1 (FeN), closer to 8.2 Å −1 observed from the Fe foil. All these analyses confirm that the Fe 3 N structure has more metal character than the FeN structure. Fig. 2: Fe-N NP coordination and electron structure characterization. a The normalized Fe K-edge EXAFS spectra. Inset: the local FeN structure showing tetrahedral coordination (right) and Fe 3 N structure showing octahedral coordination (left). b Fe K-edge FT-EXAFS in R space and c wavelet transforms for the k 3 -weighted EXAFS signals for FeN, FeN/Fe 3 N, Fe 3 N, and Fe foil. d The N 1 s XPS spectra, e the normalized area of Fe–N bond, f the Fe 2 p XPS spectra, and g the normalized area of Fe 3+ /Fe 1+ for FeN, FeN/Fe 3 N, and Fe 3 N, respectively. Full size image The Fe–N network structure was characterized by Raman spectroscopy (Supplementary Fig. 11 ). The same D and G peak position with slightly different I D /I G values (1.26 for FeN/Fe 3 N, 1.15 for FeN, and 1.21 for Fe 3 N) suggest that more defects exist in the FeN/Fe 3 N structure [32] , which supports what is concluded from the BET N 2 -adsorption analysis. X-ray photoelectron spectroscopy (XPS) shows that the NP sample contains C (C 1 s spectra at 284.6 eV, Supplementary Fig. 12 ) and three different N’s (N 1 s spectra, Fig. 2d ) [33] . The FeN/Fe 3 N interface structure has the largest Fe–N bonding area (Fig. 2e ). Two spin-orbit doublets of Fe 2 p can be found in Fe 2 p spectra (Fig. 2f ). The Fe 2 p 3/2 peaks shift from 711.3 eV (for FeN) to 708.6 eV (for Fe 3 N) while the peak for the FeN/Fe 3 N interface structure locates at 710.3 eV, indicating that the Fe valence state in the FeN/Fe 3 N structure is between FeN and Fe 3 N and electrons are drawn from Fe 3 N to FeN. Comparing with the normalized Fe−N bonding area for FeN and Fe 3 N, we calculated that the FeN/Fe 3 N interface structure contained 66% FeN and 34% Fe 3 N (Fig. 2g ). The Fe binding environment was finally characterized by Mössbauer spectroscopy [34] , [35] , as shown in Supplementary Fig. 13 . The fitting matches well with the experimental spectra, indicating that the FeN, FeN/Fe 3 N, and Fe 3 N structures have the Fe−N 4 , Fe−N 4 /Fe−N 2 , and Fe−N 2 coordination, respectively. The electrocatalytic performance of these Fe−N NP catalysts for CO 2 RR was evaluated by linear scan voltammetry (LSV, Supplementary Fig. 14 ) and cyclic voltammetry (CV, Supplementary Fig. 15 ) in an H-type cell filled with the Ar- and CO 2 -saturated 0.5 M KHCO 3 electrolyte at room temperature [36] , [37] . The FeN/Fe 3 N structure is more responsive to the voltammetry tests, showing higher current density than either the FeN or Fe 3 N structure, suggesting that it initiates more CO 2 RR. Under a constant reduction potential, CO 2 RR products were characterized by gas chromatograph (GC) and nuclear magnetic resonance (NMR). In the current electrocatalytic reaction condition, the FeN/Fe 3 N structure is the most active catalyst for reducing CO 2 to CO with the CO formation FE reaching 98% at −0.4 V and above 90% at −0.5 to −0.9 V (Fig. 3a ). The H 2 was another gas product (Supplementary Fig. 16 ) and no liquid products were detected (Supplementary Fig. 17 ). 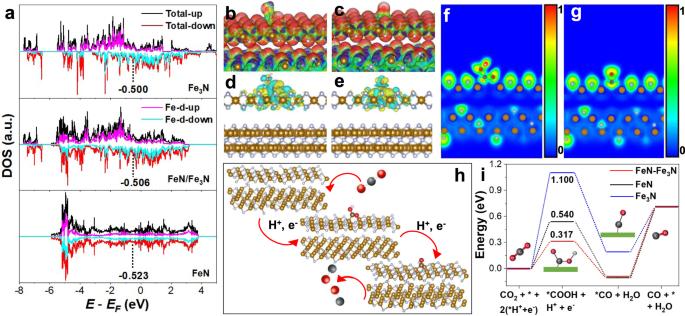Fig. 5: DFT calculations on the Fe−N catalyzed CO2RR. aThe electronic density of states and d-band centers of Fe in the FeN, Fe3N, and FeN/Fe3N structures. The electrostatic potential for adsorption of COOHband COcon the FeN/Fe3N interface. 3D electron density difference distributions for adsorption of COOHdand COeon the FeN/Fe3N interface. The electron localization for adsorption of COOHfand COgon the FeN/Fe3N interface.hSchematic reaction CO2RR to CO pathway projected on the FeN/Fe3N surface.iThe calculated Gibbs free energy diagrams for CO2RR on the FeN, Fe3N, and FeN/Fe3N surfaces. The FeN/Fe 3 N catalyst shows excellent CO selectivity compared with the recently reported catalysts (Supplementary Table 5 ). When the reduction potential more negative than −0.9 V, more HER was observed, which was further confirmed by DFT calculations that the H desorption energy was more than 0.9 eV on the FeN/Fe 3 N surface (Supplementary Fig. 18 ). This is also consistent with what was observed previously on *H binding energy increase at high potentials on Fe−N-based catalyst surfaces [24] , [38] . Based on the GC data from the closed reaction system, the single-pass CO 2 conversion [39] reached up to 56% at −0.8 V (Fig. 3b ). The FeN/Fe 3 N catalyst is much more selective than N doped KJ carbon (CO FE is <20%), FeN (CO FE peaks at ~80% at −0.6 V) and Fe 3 N (CO FE peaks at ~70% at −0.6 V) (Supplementary Fig. 19 ), which indicates that the FeN/Fe 3 N interface structure is key to this CO selectivity enhancement. Its highest CO partial current density is 21 mA cm geo −2 (Fig. 3c ) and the corresponding mass activity is 400 mA mg Fe −1 at −0.9 V, at which its turnover frequency (TOF, Supplementary Fig. 20 ) is 116 s −1 and turnover number (TON, Supplementary Fig. 20 ) is 99. The current density data were also normalized by geometric area of working electrode and CO 2 -BET area (Supplementary Fig. 21 ), all of which indicate the high catalytic performance of the FeN/Fe 3 N heterostructure. The FeN/Fe 3 N catalyst is superior to other representative Au, Ag, and M − N catalysts recently reported for catalyzing CO 2 RR to CO (Supplementary Table 5 ). The stability of the FeN/Fe 3 N catalyst was evaluated by time-dependent current change in 0.5 M KHCO 3 at different potentials −0.4, −0.6, −0.8 and −0.9 V (Fig. 3e ), which shows negligible decrease in both current density and CO FE in the 100 h testing period. It is worth to note that the CO FE stays above 90% during the tests, which is much better than the stability data obtained from other catalysts previously reported (Supplementary Table 5 ). We re-evaluated the FeN/Fe 3 N structure after the stability test. The XRD pattern (Supplementary Fig. 22a ) still shows typical FeN and Fe 3 N peaks, the NP morphology is well-maintained in the TEM image (Supplementary Fig. 22b ), and the interface structure is intact as evidenced by corresponding auto correlation and FFT images (Supplementary Fig. 22c ). The XPS spectra of Fe 2 p (Supplementary Fig. 23a ) and N 1 s (Supplementary Fig. 23b ), the EXAFS Fe K-edge spectra of the FeN/Fe 3 N (Supplementary Fig. 24a ), the pre-edge peak in Fe K-edge (Supplementary Fig. 24a ) and FT-EXAFS in R-space (Supplementary Fig. 24b ) all indicate there is no obvious valence state change on Fe in the Fe−N structures, further confirming that the FeN/Fe 3 N heterostructure is well-preserved after the stability test. Fig. 3: CO 2 RR performance of the FeN/Fe 3 N catalyst. a Reduction potential dependent FEs of CO and H 2 . b GC spectrum of the gas products upon a single pass CO 2 conversion (Inset: reduction potential dependent CO 2 conversion to CO). c CO partial current density and d corresponding mass activity. e CO 2 RR current density and CO FE changes at different reduction potentials over different electrolysis times. Error bars in a – d represent the standard deviation of three independent measurements. Full size image The evolution of the adsorbed CO 2 RR intermediates on Fe−N 4 , Fe−N 2 , and Fe−N 4 /Fe−N 2 sites was studied by in situ electrochemical spectroscopies. The in situ electrochemical impedance spectroscopy (EIS) [40] , [41] gives frequency-dependent changes of the Bode phase plots of the Fe−N-coordination sites, which is sensitive to the charge transfer and surface adsorption. The peaks of the FeN structure shift from middle frequency (10 0 − 10 2 Hz) to high-frequency (10 2 − 10 4 Hz) region (Fig. 4a ) due to the low charge transport ability of the Fe−N 4 coordination sites, while those of the Fe 3 N structure shift from high-frequency (10 2 − 10 4 Hz) to middle frequency region (10 0 − 10 2 Hz) (Fig. 4b ) due to the poor surface adsorption of CO on the Fe–N 2 coordination sites. In comparison, the FeN/Fe 3 N structure shows both FeN- and Fe 3 N-type Bode phase peaks, but these peaks shift to lower frequency (Fig. 4c ) due to the optimized surface adsorption energy and enhanced charge transport ability from FeN 3 to FeN. Fig. 4: In situ spectroscopic studies of Fe-N catalysts and CO 2 RR. a – c Bode phase plots of FeN a , Fe 3 N b , and FeN/Fe 3 N c at different reduction potentials. In situ DEMS plots showing the increased presence of CO with increased flowing CO 2 gas d and CO signal under different potentials e of the FeN/Fe 3 N-catalyzed CO 2 RR. f The in situ SEIR spectra of the FeN/Fe 3 N for CO 2 RR. Full size image We further conducted in situ differential electrochemical mass spectroscopy (DEMS) test to characterize products separated by the FeN/Fe 3 N-catalyzed CO 2 RR, from which the concentration of CO increases with the flowing CO 2 gas (Fig. 4d ), suggesting the detected CO is due to CO 2 RR. The CO signal in DEMS tests is enhanced from −0.2 to −0.8 V vs . RHE (Fig. 4e ), indicating that the CO is the main product for CO 2 RR (Supplementary Fig. 25 ). We performed in situ spectra in the CO 2 -flowed 0.5 M KHCO 3 electrolyte at various reduction potentials to characterize CO 2 reduction intermediates. The *CO and *H competition was evidenced from in situ surface enhancement infrared spectroscopy (SEIR) [42] , [43] . According to the electrochemical Stark effect [44] , [45] , the vibrational frequencies of the intermediates adsorbed on an electrode usually shift negatively. As shown in Fig. 4f , there is no peak observed at ~1900 cm −1 from open circuit voltage (OCV) to −0.2 V. However, at −0.4 V, a small peak at ~1920 cm −1 starts to appear, and shows a negative shift with 49.66 cm −1 per voltage from −0.4 to −1.2 V, which attributes to the adsorbed CO* peak [46] , [47] , [48] , [49] . At more negative potentials, the intensity of the CO peak increases initially, but starts to drop after −1.2 V due to the strong competition of H* generated from the enhanced HER [50] . From the Raman spectra (Supplementary Fig. 26a ), the electrolyte, CO 2 , CO, and H 2 O peaks can be found. The two peaks for HCO 3 − at ~1010 cm −1 and CO 3 2− at ~1060 cm −1 are found from the 0.5 M KHCO 3 electrolyte [51] , while the ~1920 cm −1 peak has a negative shift from −0.4 to −0.8 V, which corresponds to the stretching vibration mode of the adsorbed CO [45] (Supplementary Fig. 26b ). In situ Raman spectra of CO 2 adsorption peaks at ~2330 cm −1 for FeN (Supplementary Fig. 26c ), Fe 3 N (Supplementary Fig. 26d ), and FeN/Fe 3 N (Supplementary Fig. 26e ) also intensify with enhanced voltage from OCV to −0.8 V vs. RHE (Supplementary Fig. 26f ), demonstrating that the FeN/Fe 3 N heterostructure has an optimized interfacial adsorption ability. The formation of CO from CO 2 RR is generally believed to follow two proton-coupled electron-transfer steps to form COOH*, and then CO* that is desorbed from the catalyst surface [52] , [53] , [54] . In this process, the formation of COOH* usually is a potential-limiting step due to the high activation energy of CO 2 molecule. To understand the Fe−N catalysis better, we used DFT to calculate the related activation energy on the catalyst surfaces. We compared the electronic density of states (DOS) and d-band center of Fe 3 N, FeN, and FeN/Fe 3 N structures [55] , [56] , [57] . As shown in Fig. 5a , the d-band center of the FeN/Fe 3 N heterostructure is at −0.506 eV, while that of FeN is at −0.523 eV and Fe 3 N at −0.500 eV, suggesting Fe 3 N is beneficial to improve the overall d-band center shift to the Fermi level (E F ). Additionally, the d-band center of pure FeN (100), pure Fe 3 N (001), FeN cell, and Fe 3 N cell is −0.591, −0.503, −0.647, and −0.502 eV (Supplementary Fig. 27 ), further demonstrating Fe 3 N with rich electron is key for built-in electric field from Fe 3 N to FeN. As a result, the intensity of DOS (Supplementary Fig. 28 ), and the integral DOS (IDOS) (Supplementary Fig. 29 ) of the FeN/Fe 3 N structure is higher than that of the FeN or Fe 3 N structure, suggesting that electrons are more populated at E F level on the FeN/Fe 3 N surface for effective binding of reaction intermediates. The FeN/Fe 3 N surface potential change upon binding to COOH and CO was calculated by electrostatic potentials and shown as colored contours in Fig. 5b (for *COOH) and Fig. 5c (for *CO), which shows that electron transfer causes a decrease in the potential of CO and COOH (red means lower electrostatic potential and blue means higher electrostatic potential). The corresponding 3D electron density distributions on the FeN/Fe 3 N (Fig. 5d, e ), FeN (Supplementary Fig. 30c, d ), and Fe 3 N (Supplementary Fig. 31c, d ) surfaces upon their binding to COOH and CO suggest that electrons are transferred from catalyst to COOH/CO. The electron localization of COOH and CO on the FeN, Fe 3 N, and FeN/Fe 3 N surface calculated by electron localization function is about 0.8, 0.7, 0.8 (Supplementary Fig. 30e , Supplementary Fig. 31e and Fig. 5f ) for COOH and 0.7, 0.7, 0.7 (Supplementary Fig. 30f , Supplementary Fig. 31f and Fig. 5g ) for CO, indicating that COOH and CO interact covalently with the catalyst surface [58] , [59] , [60] . Following the common CO 2 RR reaction pathway specifically on the FeN/Fe 3 N surface (Fig. 5h ), we calculated the Gibbs free energy (ΔG) for the potential-limiting step (CO 2ad to *COOH) on the FeN/Fe 3 N structure to be 0.317 eV (Fig. 5i ), much lower than that on the FeN (0.540 eV) and Fe 3 N (1.10 eV) in the heterostructure. We also calculated the CO 2 RR performance on the other side of FeN/Fe 3 N heterostructure on the interface Fe 3 N (001) (Supplementary Fig. 32a ) and other side of Fe 3 N (001) (Supplementary Fig. 32b ). The ΔG for CO 2 to COOH is 0.985 eV on the interface Fe 3 N (001), ΔG for *CO on other side of Fe 3 N (001) is −2.566 eV, which is too stable for the CO to dissociate from the plane. ΔG for CO 2 to COOH is about 0.360 and 1.08 eV on the pure FeN (100) (Supplementary Fig. 32c ) and pure Fe 3 N (001) (Supplementary Fig. 32d ), indicating that CO 2 adsorption and activation on the FeN (100) is more favorable for CO 2 RR. We further constructed the FeN (110)/Fe 3 N (001) heterostructure to reveal the role of the FeN (110) plays on catalyzing CO 2 RR. The electron cloud around N and Fe in the Fe 3 N region (yellow) is much more enriched than that in the FeN region (blue) (Supplementary Fig. 33a ), while is also supported by the 2D electron localization function (Supplementary Fig. 33b ). These indicate that the FeN (110)/Fe 3 N (001) structure has no electron transport across interface and is not active for CO 2 RR. Then, the ΔG for CO 2ad to *COOH on the FeN (110)/Fe 3 N (001) structure is 1.189 eV (Supplementary Fig. 33c ) much larger than that of FeN (100)/Fe 3 N (001) heterostructure, further demonstrating that FeN (100)/Fe 3 N (001) heterostructure is superior for CO 2 RR. Our calculations support what we concluded from both structure and catalysis analysis of the Fe−N catalysts that the FeN (100)/Fe 3 N (001) interface with the built-in electric field has abundant electrons closer to E F for CO 2 adsorption and activation, showing much enhanced catalysis for CO 2 RR to CO. Fig. 5: DFT calculations on the Fe−N catalyzed CO 2 RR. a The electronic density of states and d-band centers of Fe in the FeN, Fe 3 N, and FeN/Fe 3 N structures. The electrostatic potential for adsorption of COOH b and CO c on the FeN/Fe 3 N interface. 3D electron density difference distributions for adsorption of COOH d and CO e on the FeN/Fe 3 N interface. The electron localization for adsorption of COOH f and CO g on the FeN/Fe 3 N interface. h Schematic reaction CO 2 RR to CO pathway projected on the FeN/Fe 3 N surface. i The calculated Gibbs free energy diagrams for CO 2 RR on the FeN, Fe 3 N, and FeN/Fe 3 N surfaces. Full size image In summary, we have reported a process for synthesizing heterostructured FeN/Fe 3 N NPs with the NP surface populated with Fe–N 4 /Fe–N 2 interfaces. Electron polarization from Fe 3 N (Fe−N 2 site) to FeN (Fe−N 4 site) builds the desired electric field across the FeN/Fe 3 N interface, enhancing its power to adsorb CO 2 . In the electrochemical reduction condition, this FeN/Fe 3 N structure has an excellent mass and electron transfer ability in catalyzing CO 2 RR to CO with high FE (98% at −0.4 V) and much improved stability in the 100 h electrolysis period (FE > 90% in the broad −0.4 to −0.9 V potential range). The catalyst surface adsorption of CO 2 and its activation intermediates is further characterized by various in situ spectroscopy techniques (EIS, DEMS, IR and Raman) from which the adsorbed CO* is identified. DFT calculations suggest that the FeN/Fe 3 N structure has a d-band center that is closer to its E F level where there are abundant electrons for binding to reaction intermediates (CO 2ad , COOH*, CO*). This strong interaction reduces the ΔG of the CO 2ad to COOH* conversion and provides a necessary force to lower the reduction overpotential and improve the catalytic efficiency. Our work demonstrates that creating a polarized field on the NP surface is a promising approach to the design of highly active catalysts for electrochemical CO 2 RR. Synthesis of Fe−N based precursor Firstly, the commercial Ketjen (KJ) carbon (0.1 g) was suspended in water (H 2 O, 50 mL) by ultrasound. Then, a mixture of iron (III) nitrate hexahydrate (Fe(NO 3 ) 3 •9H 2 O, 0.01 mol, 4.04 g) and urea (CH 4 N 2 O, 0.1 mol, 6.00 g) was added into the carbon suspension and continued ultrasound for 8 h. Finally, the precipitate was separated by centrifuge (6000 rpm (4830 × g ), 5 min) and washed with water and ethanol for three times and dried under vacuum at 60 °C for 6 h to give the Fe−N based precursor. Synthesis of FeN, FeN/Fe 3 N, and Fe 3 N nanosparticles 100 mg Fe−N precursor was placed in crucible and put in the tube furnace (Supplementary Fig. 1 ). Then the tube was heated to 300, 500 or 700 °C with a rate of 5 °C min −1 for 2 h under the flowing NH 3 atmosphere. Finally, the system was cooled to room temperature under a flowing NH 3 gas. In this process, FeN, FeN/Fe 3 N and Fe 3 N were obtained at 300 °C, 500 °C, and 700 °C, respectively [33] . Catalyst characterization X-ray diffraction (XRD) experiments were conducted from 20° to 90° on an X’Pert ProX-ray diffractometer with Cu Ka radiation (λ = 0.1542 nm) under a voltage of 40 kV and a current of 40 mA. Sample compositions were determined by ICP-AES (HITACHI P-4010, Japan). Product morphology was imaged by field-emission scanning electron microscopy (FESEM, Zeiss) at an acceleration voltage of 5 kV. All samples were coated with a thin layer of gold prior to FESEM observations. More detailed product morphology and structure were analyzed by transmission electron microscopy (TEM) and high-resolution transmission electron microscopy (HRTEM) under an acceleration voltage of 200 kV with a JEOL JEM 2100 TEM. Atomic-scale STEM images were recorded on a probe aberration-corrected STEM (Cubed Titan G2 60-300, FEI, USA) operated at 300 kV. Product surface composition was analyzed by X-ray photoelectron spectroscopy (XPS) with a VG ESCALAB 220I-XL device. All XPS spectra were corrected using C1 s line at 284.6 eV. The absorption spectra of Fe K-edge were collected in transmission mode using a Si (111) double-crystal monochromator at the BLW141 station of the Beijing Synchrotron Radiation Facility (BSRF). Transmission 57 Fe Mössbauer spectra were recorded by using a conventional spectrometer working in constant acceleration mode. A 50 mCi of 57 Co embedded in a Rh matrix moving at room temperature was used as the γ-ray source. The absorber was prepared with a surface density of ~8 mg cm −2 natural iron. The drive velocity was calibrated with sodium nitroprusside at room temperature and all the isomer shifts quoted in this work are relative to that of the α-Fe. Lattice mismatch calculation The lattice mismatch for the heterostructure can be calculated by lattice of different domains, as shown below: 
    δ=(2×|a_1-a_2|)/(a_1+a_2)
 (1) where δ is lattice mismatch, a 1 and a 2 are the lattice parameters of different domains. We define that two lattices are well-matched when δ is < 5%, semi-matched if δ is between 5% and 25%, and totally mismatched if δ is >25%. The δ value for the FeN/Fe 3 N heterostructure is 5.12% ( δ FeN/Fe3N = (2 × |a FeN – a Fe3N | )/(a FeN + a Fe3N ) = (2 × |0.19 – 0.20 | )/(0.19 + 0.20) = 5.12%), therefore, the FeN and Fe 3 N lattices are well-matched, which is favorable for electron transfer at the interface. Electrochemical test for CO 2 RR Electrochemical measurements were carried out at room temperature using the three-electrode system directly connected to a CHI 760 E Electrochemical Workstation (CHI Instruments, Shanghai Chenhua Instrument Corp., China). The CHI workstation was used to conduct CO 2 reduction experiments in aqueous 0.5 M KHCO 3 (pH = 6.8 when saturated with CO 2 , pH = 8.3 when saturated with Ar). A platinum wire was used as counter electrode. All potentials were measured against an Ag/AgCl reference electrode (4.0 M KCl, Pine instrument) and were calibrated against a reversible hydrogen electrode (RHE). The experiments were performed in a gas-tight cell with two-compartments separated by an anion exchange membrane (Nafion® 212). Each compartment contained 10 mL electrolyte with approximately 10 mL headspace [6] , [37] . Product analysis CO 2 gas was delivered at an average rate of 30 mL min −1 (at room temperature and ambient pressure) and routed directly into the gas sampling loop of a gas chromatograph (Agilent 7890 A). The gas phase composition was analyzed by GC every 30 min. The GC analysis was set up to split the gas sample into two aliquots whereof one aliquot was routed through a packed MoleSieve 5 A column and a packed HP-PLOT Q column before passing a thermal conductivity detector (TCD) for H 2 quantification. Argon (Corp Brother, 99.9999%) and Helium (Corp Brother, 99.9999%) were employed as carrier or make-up gases respectively. The second aliquot was routed through a packed HP-PLOT Q + PT column equipped with a flame ionization detector (FID) for analyzing CO and C 1 to C 3 hydrocarbons. The GC was calibrated using commercially available calibration standards from JJS Technical Services. 1 H-NMR spectroscopy was employed to characterize and quantify CO 2 reduction products at the end of the experiments. 1 H-NMR spectra were recorded on Bruker DRX 400/600 Avance. A total of 0.5 ml electrolyte and 0.1 ml D 2 O (content 0.05 μL dimethyl sulfoxide (DMSO), as inner standard) were mixed together to get the NMR signal. Theoretical calculations The first-principles density functional theory (DFT) calculations were performed within the generalized gradient approximation (GGA) based on via Vienna abinitio simulation package (VASP) [61] , [62] , [63] . We constructed FeN/Fe 3 N interface structure, FeN and Fe 3 N surface model with periodicity in the x and y directions and the depth of the vacuum layer is greater than 20 Å in order to prevent self-interactions. In addition, the bottom two stoichiometric layers were need to be fixed while the top layer and adsorbates (CO*, COOH*) were allowed to relax in the optimization of the FeN/Fe 3 N and Fe 3 N, for FeN, only one stoichiometric layer needs to be fixed. The VASP was employed to perform all DFT calculations within the functional as proposed by Perdew-Burke-Ernzerh (PBE) [61] , [64] of interactions is represented using the projector augmented wave (PAW) [61] , [65] , [66] potential. The Kohn-Sham one-electron valence states were expanded on the basis of plane waves with a cutoff energy of 400 eV in the in the process of structure optimization. A geometry optimization was considered convergent when the electronic energy and Hellmann-Feynman forces convergence criterion was smaller than 10 −5 eV and 0.03 eV Å −1 , respectively. The K-point of 3 × 1 × 1 was used for the optimization of the FeN/Fe 3 N, FeN and Fe 3 N surface, and the corresponding adsorption structure (CO*, COOH*). Subsequently, we calculated the charge density, electron localization function (ELF), work function and electrostatic potential in the self-consistent process. The electronic energy was considered self-consistent while the energy variation was smaller than 10 −5 eV. The value of K-point, cutoff energy is the same as the process of structure optimization. After the self-consistent calculation converges, the charge density distribution, electron localization, electrostatic potential and work function can be obtained, the self-consistent structure is used as the input file, and the wave function and charge density file are read to obtain the density of states of the heterojunction, FeN and Fe 3 N. The d-band center was used to understand the adsorption capacity of the different catalyst (FeN/Fe 3 N, FeN and Fe 3 N) surface for CO 2 . The calculation formula of d-band center: 
    ε_d=∫_-∞^∞n_d(ε )ε dε/∫_-∞^∞n_d(ε )dε
 (2) where nd(ɛ) represents the density of states and ɛ represents the energy of state. The Gibbs free energy also was calculated in this study. The zero-point energy (ZPE) correction was performed referring to the approaches previously reported. In the DFT process, we calculated the Gibbs free energy according to the equations as follow: [61] 
    G^0=E_DFT+ZPE-TS^0
 (3) Where G 0 is the Gibbs free energy, E DFT is total free energy, ZPE is the vibration energy; TS 0 is the entropy change (T = 298.15 K). TOF and TON calculation for FeN/Fe 3 N catalyst The turnover frequency (TOF) was calculated by the following formula: [67] 
    TOF=j×S×FE/2×n×F
 (4) where j (mA cm −2 ) is the current density at −0.4 V, S is the surface area of the working electrode, FE is the Faraday efficiency of CO, the number 2 means 2 electrons mol –1 of CO, F is Faraday’s constant (96485.3 C mol –1 ), and n is the moles of coated Fe atoms on the electrode. The Fe content of catalysts was measured by the ICP-AES measurement. Similarly, the turnover number (TON) of the catalyst was calculated based on: 
    TON=TOF×FE× 0.01
 (5)